Divergent sorting of a balanced ancestral polymorphism underlies the establishment of gene-flow barriers inCapsella In the Bateson–Dobzhansky–Muller model of genetic incompatibilities post-zygotic gene-flow barriers arise by fixation of novel alleles at interacting loci in separated populations. Many such incompatibilities are polymorphic in plants, implying an important role for genetic drift or balancing selection in their origin and evolution. Here we show that NPR1 and RPP5 loci cause a genetic incompatibility between the incipient species Capsella grandiflora and C. rubella , and the more distantly related C. rubella and C. orientalis . The incompatible RPP5 allele results from a mutation in C. rubella , while the incompatible NPR1 allele is frequent in the ancestral C. grandiflora . Compatible and incompatible NPR1 haplotypes are maintained by balancing selection in C. grandiflora , and were divergently sorted into the derived C. rubella and C. orientalis . Thus, by maintaining differentiated alleles at high frequencies, balancing selection on ancestral polymorphisms can facilitate establishing gene-flow barriers between derived populations through lineage sorting of the alternative alleles. Speciation proceeds by the establishment of barriers to gene-flow between different populations, ultimately resulting in reproductive isolation [1] . Gene-flow barriers can act at the prezygotic stage, for example, by restricting the temporal overlap of the reproductive periods, or at the post-zygotic stage, by decreasing the fitness of hybrid progeny. Such post-zygotic barriers to gene flow often result from the establishment of Bateson–Dobzhansky–Muller incompatibilities (BDMIs) [1] , [2] , [3] , [4] . According to this model, novel alleles at one or more loci become fixed in separated populations, either due to genetic drift or selection, and produce detrimental consequences when combined in hybrid offspring after crossing [2] . Several loci causing BDMIs have been isolated from plant and animal species [3] , [5] . In plants, an autoimmune response termed hybrid necrosis represents a prominent manifestation of BDMIs [6] , [7] , [8] , [9] , [10] , [11] , [12] , [13] . Hybrid-necrosis results from the constitutive activation of the plant immune response due to a mismatch between different allelic versions of proteins involved in the response to pathogen infection. In particular, a comprehensive analysis of hybrid-necrosis cases within Arabidopsis thaliana has highlighted the family of nucleotide-binding leucine-rich repeat (NB-LRR) proteins as particularly prone to giving rise to hybrid necrosis [14] . NB-LRR proteins activate immune responses after detecting specific pathogen-derived proteins or their effects on host proteins and are highly variable between different genotypes [15] , [16] . Despite this progress in identifying causal BDMI genes, the evolutionary history and potential selection acting on incompatible alleles remain incompletely understood. In particular, the observation that in contrast to animals, many BDMIs are polymorphic within plant species, with segregating compatible and incompatible alleles at the causal loci, suggests a greater role for either genetic drift and/or balancing selection in the origin of BDMIs in plants than in animals [4] , [5] ; however, the relative role of drift versus balancing selection remains uncertain. One scenario where polymorphic alleles may make an important contribution to the establishment of gene-flow barriers is speciation associated with the transition from outbreeding to selfing, which has occurred many times independently in flowering plants [17] . Transitions to selfing entail a loss of heterozygosity, low effective population sizes and often genetic bottlenecks in the selfing populations. This can lead to a loss of both neutral and selected polymorphisms, thereby converting standing variation into fixed differences between different selfing populations [17] . Once fixed for alternative, functionally differentiated alleles, only one novel incompatible mutation to an interacting locus would be required to establish a BDMI between the derived populations [5] . This scenario could explain the observation that the transition to selfing appears to accelerate the establishment of post-zygotic gene-flow barriers between different selfing lineages and with the ancestral outbreeding species [17] , [18] , [19] , [20] . The genus Capsella provides a tractable experimental system for testing competing models of the evolution of BDMIs associated with the transition to selfing. Within the last 100,000 years, the predominantly self-fertilizing C. rubella evolved from the outbreeding ancestor C. grandiflora via break-down of self-incompatibility and an associated severe genetic bottleneck [21] , [22] , [23] . An earlier speciation event ∼ 840,000 years ago [24] gave rise to C. orientalis , which experienced an independent transition to selfing, from a presumed C. grandiflora -like ancestor [25] . While C. grandiflora is largely restricted to Greece, C. rubella is found around the Mediterranean and beyond, and C. orientalis occurs in Central Asia [25] . C. grandiflora and C. rubella co-occur in Greece, with more recent gene flow between them [26] . Here we exploit this system to show conclusively that a gene underlying a polymorphic BDMI is maintained as polymorphic by balancing selection in the ancestral outcrosser C. grandiflora . Independent transitions to selfing have led to the fixation of alternative alleles in the derived selfers C. rubella and C. orientalis , contributing to a genetic incompatibility between them. A two-locus, immune-related incompatibility in Capsella To determine whether genetic incompatibilities exist between the recently diverged Capsella species, we analysed a C. grandifora × C. rubella recombinant inbred line (RIL) population [27] for incompatible phenotypes. In 13.3% of the RILs (19 of 142), we observed strongly retarded growth and severe stunting ( Fig. 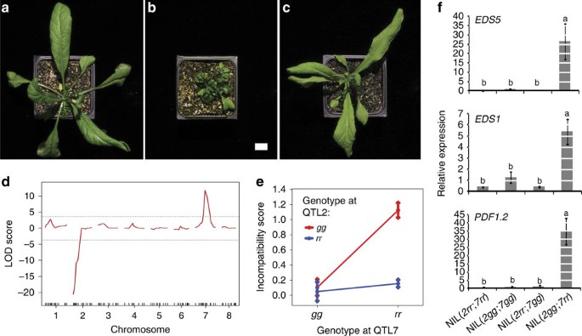Figure 1: Incompatibility betweenC. grandifloraandC. rubelladue to a constitutive immune response. (a)C. rubella, (b) incompatibleC. grandiflora×C. rubellaRIL hybrid and (c)C. grandifloraplant. Scale bar, 1 cm. (d) QTL mapping for stunted growth in the RIL population (n=142). LOD scores are multiplied by the sign of the additive effect of the locus. Dashed line represents the genome-wide 5% significance threshold. (e) Interaction plot ofgrandiflora(g) andrubella(r) alleles at QTL2 and QTL7. Incompatibility scores were determined based on visible inspection of phenotypes. Values correspond to the means±s.e.m forn=21, 18, 9 and 78 for the genotype groups (2gg;7gg),(2rr; 7gg), (2gg; 7rr) and (2rr; 7rr), respectively. (f) Expression of immune-response genes determined by quantitative reverse transcription–PCR normalized toCapsella TUB6. Mean±s.e.m. of three biological replicates is shown. Letters indicate significant differences as determined by Tukey’s honest significant difference test (α=0.05). Means belonging to the same group, as indicated by the same letters, are not significantly different. 1a–c , Supplementary Table 1 ). Quantitative trait locus (QTL) mapping identified two major QTL on chromosomes 2 and 7 as responsible for the growth defect ( Fig. 1d , Supplementary Fig. 1a ). Plants homozygous for the grandiflora allele at QTL2 ( 2gg ) and for the rubella allele at QTL7 ( 7rr ) display a reduced biomass, indicating a strong negative epistatic interaction between these loci ( Fig. 1e , Supplementary Fig. 1b ). 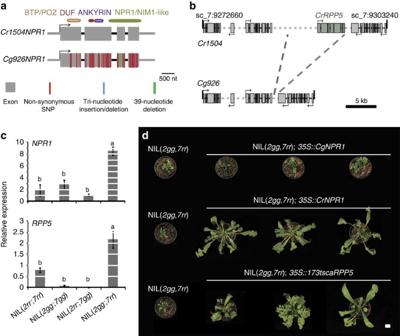Figure 2: Genetic basis of the incompatibility betweenC. grandifloraandC. rubella. (a) Gene structure, location of functional domains and polymorphisms betweenC. grandifloraandC. rubella NPR1alleles from the RIL population. Rectangles are coding sequence, lines are untranslated regions and introns. (b) Gene structure and genomic organization ofRPP5region from the RIL parents. Rectangles and solid lines are exons and introns; dashed line represents intergenic sequence. (c) Expression ofNPR1andRPP5determined by quantitative reverse transcription–PCR normalized toCapsella TUB6. Mean±s.e.m. of three biological replicates is shown. Letters indicate significant differences as determined by Tukey’s honest significant difference test (α=0.05). Means belonging to the same group, as indicated by the same letters, are not significantly different. (d) Rescue of incompatible phenotype by suppression ofRPP5expression (bottom) and by transgenic expression of theCrNPR1(middle), but not of theCgNPR1allele (top). Scale bar, 1 cm. To validate the QTL mapping results, we generated near-isogenic lines (NILs) segregating for the two QTL regions in an otherwise largely C. rubella -derived background ( Supplementary Table 2 ). Analysis of these NILs confirmed the incompatibility in 2 gg; 7rr plants ( Supplementary Fig. 1b ). While the incompatible grandiflora QTL2 allele was fully recessive, the rubella QTL7 allele was semi-dominant ( Supplementary Fig. 1b ). We focussed our subsequent analysis on these NILs, as no suitable inbred lines are available for the obligate outbreeder C. grandiflora ; as a result, genetic background variation between C. grandiflora individuals could confound any comparisons between the parental species and the NILs. Figure 1: Incompatibility between C. grandiflora and C. rubella due to a constitutive immune response. ( a ) C. rubella , ( b ) incompatible C. grandiflora × C. rubella RIL hybrid and ( c ) C. grandiflora plant. Scale bar, 1 cm. ( d ) QTL mapping for stunted growth in the RIL population ( n =142). LOD scores are multiplied by the sign of the additive effect of the locus. Dashed line represents the genome-wide 5% significance threshold. ( e ) Interaction plot of grandiflora (g) and rubella (r) alleles at QTL2 and QTL7. Incompatibility scores were determined based on visible inspection of phenotypes. Values correspond to the means±s.e.m for n =21, 18, 9 and 78 for the genotype groups (2 gg;7gg), (2 rr; 7gg), ( 2 gg; 7rr ) and (2 rr; 7rr) , respectively. ( f ) Expression of immune-response genes determined by quantitative reverse transcription–PCR normalized to Capsella TUB6 . Mean±s.e.m. of three biological replicates is shown. Letters indicate significant differences as determined by Tukey’s honest significant difference test ( α =0.05). Means belonging to the same group, as indicated by the same letters, are not significantly different. Full size image At the cellular level, reduced leaf growth in affected hybrids was largely caused by impaired cell expansion ( Supplementary Fig. 1c ). Several similar genetic incompatibilities segregating within A. thaliana result from an ectopic autoimmune response including necrosis [8] , [13] . While the incompatible Capsella hybrids did not show any ectopic cell death ( Supplementary Fig. 2b ), expression of ENHANCED DISEASE SUSCEPTIBILITY 1 ( EDS1 ) and EDS5 is strongly upregulated in incompatible hybrids ( Fig. 1f ); both genes are required for the accumulation of the plant hormone salicylic acid and establishment of systemic acquired resistance in a feed-forward loop [28] , [29] , [30] . Expression of the jasmonate- and ethylene-responsive gene PLANT DEFENSIN 1.2 (ref. 31 ) was also upregulated, in contrast to several other markers of an activated pathogen response ( Supplementary Fig. 2a ). As in A. thaliana [13] , the stunted growth resulting from this autoimmune response could be suppressed by growth at high temperature ( Supplementary Fig. 2c ). Thus, a two-locus, negative epistatic interaction causes symptoms resembling a constitutive activation of the immune response and stunted growth in C. grandiflora × C. rubella hybrids. Identification of incompatibility loci Fine mapping in the segregating NIL progeny localized the causal gene underlying QTL2 to a 40-kb interval containing the Capsella orthologue of the immune-response factor NON-EXPRESSOR OF PR-GENES1 ( NPR1 ; ref. 32 ) ( Fig. 2a ; Supplementary Fig. 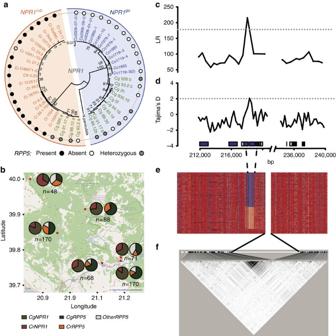Figure 3: Balancing selection maintains functionally divergent haplotypes atNPR1. (a) Phylogeny ofNPR1alleles based on a 700-bp fragment fromC. grandiflora(green),C. rubella(orange) andC. orientalisaccessions (blue). DifferentNPR1alleles from the same heterozygousC. grandifloraaccession are indicated by ‘a’ and ‘b’ after accession name. The incompatibleNPR1allele from theCg926parent of the RIL population is termed ‘926b’. Presence or absence ofRPP5is indicated. (b) Allele frequency distribution at theNPR1andRPP5loci within naturalC. grandiflorapopulations.CrRPP5andCgRPP5indicate the frequency of theCr1504 RPP5and theCg926 RPP5alleles, respectively. ‘OtherRPP5’ indicates the frequency of individuals, where none of these two alleles could be amplified. The sample size for each population is indicated on the figure under each pie chart (n). The map is based on OpenStreetmap (https://www.openstreetmap.org/copyright). (c,d) Composite likelihood ratio (LR) test of selection in 50-SNP windows (d) and estimates of Tajima’s D in 500 bp windows with 250 bp overlaps (d) from 178 resequencedC. grandifloraindividuals. Dashed line shows the 99.9% percentile across chromosome 2 as the genomic control. (e) Haplotype structure in the region surroundingNPR1in the 178C. grandifloraindividuals. For each called variant, red indicates the sample is homozygous for theC. rubellareference allele, pink is heterozygous and blue is homozygous for the alternate allele. (f) Pairwise linkage disequilibrium between variants across the region. Black: r2=1, white: r2=0. Gaps inc–fare due to missing data after filtering in a 13.7-kb interval. 3a ; Supplementary Table 3 ). NPR1 is a central regulator of systemic acquired resistance, a systemic response to pathogen infection that does not induce cell death, but leads to an increase in salicylic acid content, which in turn upregulates EDS1 and EDS5 expression [28] , [29] , [30] , similar to the incompatible phenotype in Capsella . Expression analysis indicated that NPR1 was not robustly differentially expressed between NIL( 2rr; 7rr ) and NIL( 2gg; 7gg ) plants ( Fig. 2c ), suggesting that the incompatibility is due to differences in the coding sequence. To test this, incompatible NIL( 2gg; 7rr ) plants were transformed with constructs for constitutive expression of the C. rubella NPR1 complementary DNA (cDNA; 35S::CrNPR1 ) or the C. grandiflora NPR1 cDNA ( 35S::CgNPR1 ). While the latter had little effect on the morphological phenotype despite very high expression levels, expression of 35S::CrNPR1 abolished the stunted growth of NIL( 2gg; 7rr ) plants ( Fig. 2d ; Supplementary Fig. 3c,d ). At the gene-expression level, 35S::CrNPR1 transgenic plants showed a strong reduction in expression of the marker genes EDS1 , EDS5 and PDF1.2 ( Supplementary Fig. 3i–k ); expression of these markers was also reduced in 35S::CgNPR1 transgenic plants, albeit to a lesser extent for EDS1 and EDS5 , suggesting that the very high-level expression of CgNPR1 in the two assayed lines (2 and 3 in Supplementary Fig. 3c–k ) can partially uncouple the enhanced defence-gene expression from the stunted growth in the incompatible hybrids. We conclude that the NPR1 gene represents the incompatibility locus on chromosome 2, and the causal difference(s) between the two alleles appears to affect the encoded proteins. The two alleles show a high level of diversity within the NPR1 coding sequence with 77 non-synonymous substitutions, 3 single-codon insertions/deletions and a larger deletion of 39 nucleotides in the grandiflora allele ( Fig. 2a ; Supplementary Fig. 4b ). Figure 2: Genetic basis of the incompatibility between C. grandiflora and C. rubella . ( a ) Gene structure, location of functional domains and polymorphisms between C. grandiflora and C. rubella NPR1 alleles from the RIL population. Rectangles are coding sequence, lines are untranslated regions and introns. ( b ) Gene structure and genomic organization of RPP5 region from the RIL parents. Rectangles and solid lines are exons and introns; dashed line represents intergenic sequence. ( c ) Expression of NPR1 and RPP5 determined by quantitative reverse transcription–PCR normalized to Capsella TUB6 . Mean±s.e.m. of three biological replicates is shown. Letters indicate significant differences as determined by Tukey’s honest significant difference test ( α =0.05). Means belonging to the same group, as indicated by the same letters, are not significantly different. ( d ) Rescue of incompatible phenotype by suppression of RPP5 expression (bottom) and by transgenic expression of the CrNPR1 (middle), but not of the CgNPR1 allele (top). Scale bar, 1 cm. Full size image The causal gene underlying QTL7 was mapped to a 120-kb interval that contains the closest Capsella homologue to the TIR-NB-LRR pathogen-response regulators RECOGNITION OF PERONOSPORA PARASITICA 5 ( RPP5 ; ref. 33 ) and BAL/SUPPRESSOR OF NPR1-1,CONSTITUTIVE1 ( BAL/SNC1 ; refs 34 , 35 ) ( Fig. 2b ; Supplementary Fig. 3a ; Supplementary Table 3 ). While the gene is present in the C. rubella allele, it is deleted from the specific C. grandiflora allele segregating in the RIL population ( Fig. 2b ). To test the role of CrRPP5 in causing the incompatible phenotype, its expression was reduced in incompatible NIL( 2gg; 7rr ) plants by specific miRNA-induced gene silencing [36] ; this was sufficient to suppress their growth defect and the constitutive defence-gene expression ( Fig. 2d ; Supplementary Fig. 3c,e–k ). Thus, an incompatibility between the grandiflora NPR1 and the rubella RPP5 alleles underlies the constitutive immune response and growth retardation in the affected hybrids. Both NPR1 and RPP5 showed higher expression levels in incompatible NIL plants than in compatible genotypes ( Fig. 2c ); for NPR1 and to a lesser extent for RPP5 , this enhanced expression was suppressed in the rescued 35S::CrNPR1 and RPP5 knock-down transformants ( Supplementary Fig. 3g,h ), suggesting that positive feed-back from the constitutive immune response is responsible for their elevated expression in the incompatible NIL plants. As RPP5 homologues in A. thaliana have been identified as strongly overrepresented among loci causing hybrid necrosis [14] , our findings suggest that their propensity for giving rise to incompatible alleles is an evolutionarily more wide-spread phenomenon that can give rise to between-species incompatibilities. Evolutionary history of the incompatible alleles To gain insights into the evolutionary history of the incompatible alleles, we sequenced an ∼ 700-bp fragment surrounding the 39-nt deletion in NPR1 from 10 grandiflora , 18 rubella and 10 orientalis accessions. The resulting gene phylogeny was split into two distinct clades almost as distant from each other as from the outgroup Neslia paniculata NPR1 sequence [37] ( Fig. 3a ; Supplementary Fig. 5a ). One clade contained all of the C. rubella and some of the C. grandiflora alleles (termed NPR1 rub ), while the other contained the remaining C. grandiflora alleles, including the incompatible one from our RIL population (allele Cg926b in Fig. 3a ), and all C. orientalis alleles (termed NPR1 go ). While overall NPR1 go alleles are somewhat closer to other Brassicaceae sequences than NPR1 rub alleles, all NPR1 go alleles contain the derived 39-nt deletion not found in other Brassicaceae species ( Supplementary Fig. 4a,b ). Figure 3: Balancing selection maintains functionally divergent haplotypes at NPR1 . ( a ) Phylogeny of NPR1 alleles based on a 700-bp fragment from C. grandiflora (green), C. rubella (orange) and C. orientalis accessions (blue). Different NPR1 alleles from the same heterozygous C. grandiflora accession are indicated by ‘a’ and ‘b’ after accession name. The incompatible NPR1 allele from the Cg926 parent of the RIL population is termed ‘926b’. Presence or absence of RPP5 is indicated. ( b ) Allele frequency distribution at the NPR1 and RPP5 loci within natural C. grandiflora populations. CrRPP5 and CgRPP5 indicate the frequency of the Cr1504 RPP5 and the Cg926 RPP5 alleles, respectively. ‘Other RPP5 ’ indicates the frequency of individuals, where none of these two alleles could be amplified. The sample size for each population is indicated on the figure under each pie chart ( n ). The map is based on OpenStreetmap ( https://www.openstreetmap.org/copyright ). ( c , d ) Composite likelihood ratio (LR) test of selection in 50-SNP windows ( d ) and estimates of Tajima’s D in 500 bp windows with 250 bp overlaps ( d ) from 178 resequenced C. grandiflora individuals. Dashed line shows the 99.9% percentile across chromosome 2 as the genomic control. ( e ) Haplotype structure in the region surrounding NPR1 in the 178 C. grandiflora individuals. For each called variant, red indicates the sample is homozygous for the C. rubella reference allele, pink is heterozygous and blue is homozygous for the alternate allele. ( f ) Pairwise linkage disequilibrium between variants across the region. Black: r 2 =1, white: r 2 =0. Gaps in c – f are due to missing data after filtering in a 13.7-kb interval. Full size image RPP5 was present in 17 out of 18 rubella accessions and absent in all of the 10 orientalis accessions ( Fig. 3a ). In grandiflora , RPP5- presence and -absence alleles segregate irrespective of the NPR1 allele found in the accessions. The different RPP 5 haplotypes seen in C. rubella reflect a subset of the haplotype variation in the ancestral C. grandiflora ( Supplementary Fig. 5b ), and the RPP5 deletion in C. grandiflora/orientalis is evolutionarily derived, as RPP5 homologues are found in the syntenic position in all other analysed Brassicaceae genomes except for two of the three subgenomes of Brassica rapa ( Supplementary Fig. 5c ). Thus, the distribution of different NPR1 and RPP5 haplotypes indicates that at both loci ancestral polymorphisms were present before the divergence of the Western Capsella lineage, including C. grandiflora and C. rubella , and the Eastern lineage, including C. orientalis (ref. 25 ). To determine the geographical distribution of the different NPR1 and RPP5 alleles within the outbreeding C. grandiflora , we genotyped six natural C. grandiflora populations from the Zagori Mountains in Greece. All six populations segregated for the NPR1 rub and NPR1 go alleles, as well as the presence or absence of RPP5 at high frequencies ( Fig. 3b ). We asked whether segregation of different alleles at both loci within C. grandiflora was associated with the occurrence of the incompatible phenotype. However, neither progenies of plants collected from the six above populations from the wild ( n =749 progeny plants) nor offspring of controlled crosses between C. grandiflora plants heterozygous at NPR1 and for presence/absence of RPP5 ( n =504 progeny plants) showed a robust incompatible phenotype associated with the expected incompatible genotype. This absence of incompatible phenotypes despite the segregation of different alleles at both loci could reflect the activity of modifier alleles at other loci that would have been lost in C. rubella or allelic heterogeneity, with only some NPR1 go alleles or some RPP5 alleles causing incompatibility. To test for allelic heterogeneity, we crossed different C. rubella and C. grandiflora accessions and analysed the progenies ( Supplementary Fig. 6 and 7a,b ; Supplementary Discussion ). An incompatible phenotype associated with the 2gg; 7rr genotype was observed when combining the RPP5 allele from Cr1504 (the C. rubella parent of the RIL population) with any NPR1 go alleles; however, this was not seen for any other RPP5 alleles, including one from the same haplotype group as that in Cr1504 (in Cr22.5 , cross 21; Supplementary Fig. 6 ). This suggests that a novel mutation(s) in RPP5 in the Cr1504 lineage led to the incompatible allele and explains the absence of incompatible phenotypes in C. grandiflora . In three of the crosses involving C. rubella accessions other than Cr1504 (crosses 3, 9 and 10), we observed similar incompatible phenotypes to the one above, with stunted growth, increased expression of immune-response genes and suppression by high temperature ( Supplementary Figs 7b and 8a,b ). Importantly, however, these incompatibilities do not involve the RPP5 locus, but do show tight linkage to NPR1 in at least two cases (crosses 3 and 9; Supplementary Fig. 7b ; Supplementary Discussion ). Thus, mutations to more than just one interacting locus can lead to the evolution of genetic incompatibilities with one of the NPR1 haplotype groups in C. grandiflora , suggesting that the presence of highly divergent alleles in a population can facilitate the establishment of BDMIs. Balancing selection maintains divergent NPR1 haplotypes The above observations raise the question how the NPR1 polymorphism is maintained in C. grandiflora ? To address this, we analysed the NPR1 region from 178 resequenced C. grandiflora individuals from a natural population in Northern Greece [26] . This demonstrated a strong signal of balancing selection on NPR1 , with a highly significant positive peak in Tajima’s D (that is, an excess of intermediate frequency alleles) and an extreme composite likelihood ratio test score ( Fig. 3c,d ). Since both of these tests are conducted in the context of the genome-wide empirical distribution, these extreme values are unlikely to be explained by demographic effects, and instead are indicative of balancing selection. The NPR1 locus also shows an unusual haplotype structure with strong linkage disequilibrium over 85% of the coding-sequence length (positions 217,869 to 219,840 on scaffold 2; NPR1 coding sequence is from position 217,594 to 219,740) ( Fig. 3a,e,f ). This unusual haplotype structure could be due to a partial selective sweep or long-term balancing selection with recombination suppression; the latter explanation is most likely, as the haplotype diversity appears to be ancient (fourfold diversity between haplotypes is 0.115, roughly six times higher than the average genome-wide pairwise diversity [21] , [22] , [23] ). Thus, the strong differentiation between the two NPR1 haplotype groups seen in the phylogenetic tree based on the 700-bp fragment reflects the long-term maintenance of highly differentiated NPR1 haplotypes in the ancestral C. grandiflora population through balancing selection and their subsequent sorting into the two selfing species ( Fig. 3a ). A comparable analysis for RPP5 was not possible, as strong structural heterogeneity of the locus precluded precise genotype reconstruction from next-generation sequencing data. Thus, we conclude that balancing selection maintains two strongly divergent NPR1 haplotype groups. We next asked whether balancing selection on NPR1 could be due to different activities of the two allele clades in setting the basal level of immune-system activation. To test this possibility, we analysed transcriptome data for 99 C. grandiflora individuals from the same sample as above [38] . No single gene showed a statistically significant expression difference between the three NPR1 genotype groups, likely reflecting the limited statistical power of the experiment. We therefore examined overrepresented functional categories among the 1,000 genes with the lowest P values when testing for an association of gene expression and NPR1 genotype. This identified a significant overrepresentation of genes involved in pathogen response, both using MapMan analysis [39] and MASTA-based comparisons [40] with published A. thaliana microarray data ( Supplementary Fig. 9 ); in particular, genes upregulated after pathogen- or elicitor-treatment in A. thaliana tend to be more strongly expressed in C. grandiflora plants homozygous for NPR1 rub alleles than in plants homozygous for NPR1 go alleles and vice versa . This suggests a functional difference between the two allele clades in basal immune-system activation as a reason for their maintenance by balancing selection. Genetic incompatibility between C. rubella and C. orientalis The two selfing species C. rubella and C. orientalis were derived independently from a C. grandiflora -like ancestor and have fixed alternative ancestral NPR1 alleles ( Fig. 3a ). In addition, C. orientalis appears to be fixed for the absence of RPP5 ( Fig. 3a ; Supplementary Fig. 5 ). We therefore tested whether hybrids of C. rubella Cr1504 and C. orientalis would show a similar incompatibility as above. F1 plants from a cross of C. rubella Cr1504 to C. orientalis showed reduced growth, and this became more pronounced in the F2 ( Fig. 4a ; Supplementary Fig. 8c ). Genotyping demonstrated that incompatibility is associated with the NPR1 go allele and C. rubella RPP5 allele. In contrast to what was observed in C. rubella × C. grandiflora hybrids ( Supplementary Fig. 1b ), the incompatible alleles at both loci acted in a semi-dominant manner, thus establishing a robust BDMI ( Supplementary Fig. 8d ). 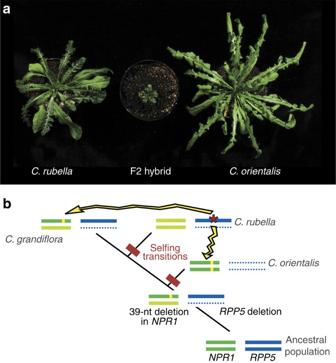Figure 4: Divergent lineage sorting of ancestral polymorphisms. (a) Plants ofC. rubella 1504,C. orientalis 1983and incompatible F2 hybrid. (b) Proposed evolutionary history ofNPR1andRPP5loci in the genusCapsella. In an ancestral population before the divergence of the three species, a deletion of theRPP5locus occurred; in addition, the 39-nt deletion occurred inNPR1(yellow box in dark greenNPR1allele) and the twoNPR1haplotype groups diverged (light and dark greenNPR1alleles). Following the independent transitions to selfing inC. orientalisandC. rubella, theNPR1haplotypes were divergently sorted;C. orientalisalso became fixed for theRPP5deletion. InC. rubella, the incompatibility-inducing mutation inRPP5arose (red asterisks), leading to BDMIs withC. grandifloraandC. orientalis(yellow arrows). Figure 4: Divergent lineage sorting of ancestral polymorphisms. ( a ) Plants of C. rubella 1504 , C. orientalis 1983 and incompatible F2 hybrid. ( b ) Proposed evolutionary history of NPR1 and RPP5 loci in the genus Capsella . In an ancestral population before the divergence of the three species, a deletion of the RPP5 locus occurred; in addition, the 39-nt deletion occurred in NPR1 (yellow box in dark green NPR1 allele) and the two NPR1 haplotype groups diverged (light and dark green NPR1 alleles). Following the independent transitions to selfing in C. orientalis and C. rubella , the NPR1 haplotypes were divergently sorted; C. orientalis also became fixed for the RPP5 deletion. In C. rubella , the incompatibility-inducing mutation in RPP5 arose (red asterisks), leading to BDMIs with C. grandiflora and C. orientalis (yellow arrows). Full size image Our results identify a negative epistatic interaction between the Capsella NPR1 and RPP5 orthologues that causes a polymorphic BDMI between the selfing C. rubella and the ancestral outbreeder C. grandiflora , as well as between the two selfing lineages C. rubella and C. orientalis . We also show that the causal NPR1 polymorphism is maintained in C. grandiflora by balancing selection, and the alternative alleles were divergently sorted into C. rubella and C. orientalis ( Fig. 4b ). How could an incompatible interaction between RPP5 and NPR1 trigger a constitutive pathogen response? NPR1 represents a central regulator of systemic acquired resistance; its salicylic acid and redox-dependent translocation into the nucleus after pathogen infection triggers large-scale transcriptional reprogramming, acting as a transcriptional co-regulator in concert with TGA-family transcription factors [30] . While overexpression of BAL/SNC1 causes a constitutive immune response and stunted growth in otherwise wild-type A. thaliana plants [34] , a constitutively active mutation in BAL/SNC1 was discovered as a suppressor of the npr1 mutant phenotype, triggering a similar phenotype even in the absence of functional NPR1 (ref. 35 ), and arguing for an NPR1 -independent role of the RPP5 -homologue SNC1 . By contrast, work in A. thaliana has also demonstrated that NPR1 function is required for race-specific downy-mildew resistance conferred by RPP5 and closely related TIR-NB-LRR proteins, highlighting a functional interaction between NPR1 and RPP5-like proteins [41] , [42] , as also suggested by our results in Capsella . However, the molecular details of this interaction have not been resolved. Our transcriptome analyses suggest that the compatible C. rubella -like NPR1 allele is more active in promoting basal resistance-gene expression than the incompatible C. grandiflora -like allele; thus, it appears unlikely that the constitutive immune response is simply triggered by the additive effect of two somewhat more active signalling molecules, whose individual effects are insufficient to trigger the response. Although there is currently no molecular evidence for such an interaction, direct binding of the incompatible protein versions to trigger an immune response is conceivable. What are the implications of our results for the evolution of BDMIs in plants? First, the compatible and incompatible NPR1 alleles in C. grandiflora provide a clear example of how balancing selection as opposed to genetic drift can underlie the frequently observed intraspecific polymorphisms for BDMIs [4] , [5] . Second, the Capsella genus demonstrates how such balanced polymorphisms can contribute to BDMIs between independently derived selfing lineages ( C. rubella and C. orientalis ), when these become fixed for the alternative alleles, likely due to stronger genetic drift in the selfing lineages. Third, it is plausible to assume that such divergent lineage sorting of functionally differentiated alleles can accelerate the establishment of BDMIs when compared with a scenario without standing variation in the ancestral population. This is because after such divergent lineage sorting only one novel incompatible mutation would be required to an interacting locus, as was the case for RPP5 in the Cr1504 lineage. Furthermore, the results from additional C. grandiflora × C. rubella crosses suggest that the NPR1 polymorphism underlies additional incompatibilities between C. grandiflora and C. rubella that involve at least one additional locus besides RPP5 . In this view, balancing selection would facilitate the evolution of BDMIs via two effects. First, the long-term maintenance of the alternative alleles would allow their higher-than-average molecular divergence, increasing the risk of incompatibilities with novel alleles at interacting loci. In the case of NPR1 , the extent of divergence between the NPR1 rub haplotypes in C. rubella and the NPR1 go haplotypes in C. grandiflora or C. orientalis is likely to be among the highest across the genome ( cf. , Supplementary Fig. 5a ); thus, mutations to genes that interact with NPR1 are more likely to give rise to an incompatibility with one of the NPR1 haplotypes than mutations at other loci that interact with genes with less divergent haplotypes. As a result, in the C. rubella lineage alleles that are incompatible with the NPR1 haplotype not found in C. rubella (that is, NPR1 go ) should arise more frequently than alleles that are incompatible with the non- C. rubella alleles at other, less divergent loci. The second effect of balancing selection would be that the balanced frequencies of the alternative alleles make their divergent lineage sorting into derived populations more likely than for more strongly skewed allele frequencies. Consistent with this notion, we note that the absence/presence polymorphism for RPP5 seen at high frequencies in C. grandiflora populations ( Fig. 3a ) appears to have undergone divergent lineage sorting into the two derived selfing species as well, with a deletion allele fixed in C. orientalis , and RPP5 presence almost fixed in C. rubella . Whether the RPP5 deletion seen in the C. rubella accession Cr1GR1-TS1 ( Fig. 3a ) reflects incomplete lineage sorting, a novel deletion in the C. rubella lineage or post-divergence introgression of a deletion allele from C. grandiflora is currently unclear. More generally, incompatibilities originating from standing variation may be also more likely to arise from loci under balancing selection than loci subject to mutation-selection balance, since their historical maintenance at higher frequencies by selection (for example, frequency-dependent selection, spatially or temporally varying selection, genotype × environment interactions) implies that both alleles can be selectively favoured under certain conditions. In contrast, alleles under mutation-selection balance are likely to be at lower initial frequencies, deleterious, and selected against. Even though it was not possible to resolve the different RPP5 haplotypes in the resequenced C. grandiflora population, most likely due to substantial structural variation, we can assume that the same evolutionary forces act on this R gene as have been described for R genes in other plant species. R genes from natural populations generally show the highest levels of genetic variation in plant genomes and evidence of balancing or diversifying selection with maintenance of polymorphisms [15] , [43] . Thus, novel R -gene alleles appear to enter and rise to appreciable frequencies in populations more often than novel alleles at other, non- R genes; at the same time, they appear to be more likely to be maintained as polymorphisms, rather than becoming fixed in the populations [15] , [43] . In the case of Capsella , this should further promote the establishment of genetic incompatibilities involving NPR1 and interacting R -genes, yet should delay or prevent fixation of incompatible R -gene alleles. At present, it is unclear how large a contribution the studied BDMI between NPR1 and RPP5 has made to speciation in Capsella , given its largely recessive behaviour and polymorphism between C. rubella and C. grandiflora , and the biogeography and evolutionary history of the C. orientalis versus the C. grandiflora / C. rubella lineages [25] . However, despite this uncertainty it suggests a potentially more wide-spread importance for ancestral polymorphisms under balancing selection as a basis for the evolution of plant BDMIs, particularly when combined with divergent lineage sorting after a transition to selfing or other genetic bottlenecks. In fact, the evolution of male semi-sterility in hybrids of japonica and indica rice supports a broadly similar scenario [44] , [45] . The causal difference in one of the two interacting loci, a C-to-T change in SaF , is found as a trans-specific polymorphism in widely diverged rice species and segregates at intermediate frequencies in current populations of the wild rice Oryza rufipogon [44] , [45] . Though not formally demonstrated, this suggests that the two alleles have been maintained by long-term balancing selection [46] . A novel mutation to the interacting locus SaM occurred in a subpopulation of O. rufipogon , causing a BDMI in SaF − SaM − / SaF + SaM + hybrids. During rice domestication, the SaF − SaM − haplotype was preferentially retained in japonica rice, while the SaF + SaM + haplotype is prevalent in indica rice, contributing to the hybrid sterility between the subspecies. Thus, while the relative timing of events seems to differ from the Capsella example, the evolution of SaF/SaM -based hybrid sterility in rice supports a potentially important role of ancestral polymorphisms under balancing selection for the evolution of plant gene-flow barriers. Biological materials and growth conditions The geographical origins of the C. grandiflora , C. rubella and C. orientalis accessions used in this study and generation of the RIL population have been described previously [26] , [27] , [47] . Additional C. grandiflora populations were collected at the locations indicated in Supplementary Table 4 . The NIL segregating for the two incompatible loci was generated by introgressing the corresponding Cg926 alleles into a Cr1504 background by four rounds of backcrossing. Its genotype is given in Supplementary Table 2 . All the plants were grown under long day conditions (16 h light, 8 h dark) at 70% humidity with a light level of 150 μmol m −2 s −1 . As default, the temperature cycle was 22 °C during the day and 18 °C during the night. The temperature rescue experiments were conducted at the indicated temperature without any diurnal fluctuations. Molecular cloning and plant transformation The 35S::CrNPR1 and 35S::CgNPR1 constructs were generated by amplifying NPR1 open reading frames (ORFs) from NIL( 2gg; 7rr ) and NIL( 2rr; 7rr ) seedling cDNA, respectively, using the primers oAS1036 and oAS1037. After subcloning PCR products into the pGEM-T vector (Promega), the NPR1 ORFs were sequenced and transferred into the plant transformation vector ML595 (a modified version of pGPTVBAR, ref. 48 ) at a PacI site located between a cauliflower mosaic virus 35S promoter and terminator. To downregulate the expression of the CrRPP5 gene in the incompatible hybrids, a microRNA-induced gene silencing construct was generated as described [36] . A 329-bp fragment of CrRPP5 cDNA was fused to the recognition site of the miR173 through PCR amplification using the primers oAS1137 and oAS1138. The resulting PCR product, 173ts:RPP5, was digested and transferred into the PacI site of ML595 as described above. The 35S::173tsRPP5 , 35S::CrNPR1 and 35S::CgNPR1 constructs were transformed into NIL( 2gg; 7rr ) plants by floral dip [49] . Phenotypic characterization Palisade sub-epidermal cell sizes were measured as previously described [50] . Briefly, entire leaves were fixed overnight at 4 °C in formalin/acetic acid/alcohol and dehydrated through a series of 70, 80, 90 and 100% ethanol, with 5-min incubation per step. The samples were then transferred into acetone and incubated for 5 min at 95°C. Finally the samples were cleared overnight in a chloral hydrate solution (200 g chloral hydrate, 20 g glycerol and 50 ml water). For observation, the samples were mounted in the chloral hydrate solution and imaged under differential interference contrast on an Olympus BX51 microscope using an AxioCam ICc3 camera (Zeiss). These images were used to determine cell area in Image J. The presence of cell death was studied by staining whole leaves with lactophenol Trypan blue as previously described [51] . Briefly, leaves were boiled in staining solution (6 vols ethanol, 1 vol water, 1 vol lactic acid, 1 vol glycerol, 1 vol phenol, Trypan blue 0.067%) for 2 min and destained in chloral hydrate (2.5 g ml −1 ). Cleared leaves were mounted in chloral hydrate and imaged using an Olympus BX51 microscope and an AxioCam ICc3 camera (Zeiss). QTL and fine mapping QTL mapping was based on the previously described genotypes of the Cr1504 x Cg926 RILs [27] . QTL analysis and testing for genetic interaction were performed using the R/QTL package adds-on implemented in the open-source statistical software R ( http://www.R-project.org/ ) [52] , [53] . Ten plants for each of the 142 RILS were scored for the severity of the hybrid incompatibility phenotype from 0 (normal growth) to 3 (strongly stunted growth). LOD scores were calculated with the Multiple QTL Mapping (MQM) function of the R/QTL package using the phenotypic mean value for each RIL and assuming a normal distribution of the phenotypic values. An unsupervised cofactor selection through backward elimination using a cofactor significance of 0.015 was conducted to identify informative markers that needed to be accounted for in the model of the MQM scan. Genome-wide permutations (1,000 permutations) were used to assess the LOD significance threshold ( α =0.05). The two-LOD score interval was used to determine the position of each QTL within 95% confidence. Additive effect and the percentage of variance explained by each QTL were determined using the fitqtl function with the formula: y ∼ Q1+Q2+Q1:Q2. The effect of the interaction between the two QTL was visualized using the effectplot R function. Genetic interactions between the QTL identified were tested using the scantwo function with an Haley–Knott regression. The PCR-based markers used for fine mapping were retrieved from the whole genome resequencing of Cr1504 and Cg926 ( Supplementary Table 5 ). The genetic mapping of the genes underlying QTL2 and QTL7 was performed using NIL( 2rg; 7rr ) and NIL( 2gg; 7rg ) plants, respectively. The progenies of these plants were screened for recombination breakpoints between the markers HiB1 and HiB8 and between HiG1 and HiG6, respectively. In total 667 and 1,117 plants were screened to narrow down the region underlying the QTL2 and QTL7. For critical recombinants, the genotype at the incompatible locus was verified by studying the segregation of the stunted growth within their progenies. Quantitative reverse transcription–PCR Total mRNA was extracted from young leaves of 20-day-old seedling, using trizol (Life Technologies), treated with Turbo DNAase (Ambion) and reverse transcribed with the Superscript III Reverse Transcriptase (Invitrogen). This template was then used to quantify relative abundance of specific transcripts using the primers described in Supplementary Table 5 , the SensiMix SYBR Low-ROX kit (Bioline) and a LightCycler 480 (Roche). Each data point was based on three technical replicates each from three biological replicates. Allele frequencies, sequence and population-genetic analyses To reconstitute the phylogeny at the NPR1 and the RPP5 loci, fragments of about 700 bp and 800 bp, respectively, were resequenced in several C. grandiflora and C .rubella accessions using the primer pairs oAS1129-oAS1130 and oAS873-oAS1123. The C. orientalis sequences were retrieved from the previously described whole genome resequencing of 10 individuals [47] . The presence or absence of the RPP5 gene was tested by PCR using the primers oAS873 and oAS1123. The phylogenetic relationship between the different sequences was investigated by constructing neighbour-joining trees with MEGA5 (ref. 54 ) using maximum composite likelihood method. Haplotype networks were reconstituted using Haplotype Viewer ( http://www.cibiv.at/~greg/haploviewer ). Allele frequencies at the NPR1 and the RPP5 loci were estimated by PCR genotyping C. grandiflora populations with the primer pair oAS1129-oAS1130 for NPR1 , and oAS873-oAS1123 and oAS839-1133 for RPP5 . The primer pair oAS1129-1130 reveals a 39-nt deletion within the exon3 of NPR1 . Primer pair oAS873-oAS1123 amplifies 1.1 kb at the 3′ end of the RPP5 ORF, while oAS839-113 reveals the 7.6 kb deletion of the RPP5 gene. The C. grandiflora seeds were collected around the Zagori Mountains in Greece leaving at least 1 m between the collected plants (see ‘Biological materials and growth conditions’ section above). Four progenies of each of these plants were independently genotyped to estimated allele frequencies. The C. grandiflora populations sampled were plotted on an OpenStreetMap ( https://www.openstreetmap.org/copyright ) based map using the R package ggmap. OpenStreetMap is available under the Open Database License (ODbL) v1.0 ( http://opendatacommons.org/licenses/odbl/1.0/ ) as OA-SA. The total number of plants genotyped is indicated in Fig. 3 . Note that for the RPP5 locus, we have not been able to amplify a fragment in all of the C. grandiflora plants, which is likely due to the high sequence and structural variability at the RPP5 locus. We have called the missing fraction of haplotypes ‘other RPP ’. Of note, this effect may have lead to an overestimation of the CrRPP5 and CgRPP5 alleles, if other RPP5 alleles went undetected in heterozygous plants. The data for population-genetic analysis and association testing are a subset of a whole genome population resequencing study of within-population variation (Lee et al. , manuscript in preparation). Briefly, 178 genotypes were derived from C. grandiflora population 9 from Epiros, Zagory mountains, Greece [55] and DNA was extracted by either a CTAB-based protocol or by DNeasy Plant Mini Kit (Qiagen). We obtained whole genome sequences from each individual through 100 cycles of paired end sequencing in a Hi-seq 2000 with Truseq libraries (Illumina). Three individuals were sequenced per lane. Reads were mapped to the C. rubella reference genome [23] with Stampy v.1.0.19. After bioinformatic processing with Picard tools, we realigned reads around putative indels with GATK RealignerTargetCreator and IndelRealigner and then compressed the resulting bams with GATK ReduceReads. Raw single nucleotide polymorphism (SNP) calls were generated by joint calling of all 178 samples in GATK v2.81 UnifiedGenotyper. We subsequently followed GATK Best Practices for Variant Quality Recalibration using a high confidence subset of the raw calls generated by filtering SNPs for concordance with common variants (>0.11) in a species-wide sample of C. grandiflora [56] , as well as suspect realignments (transposable elements, centromeres, 600-bp intervals containing extreme Hardy–Weinberg deviations, 1-kb intervals that showed evidence of three or more SNPs in a reference-to-reference mapping of 150-bp-paired end reads from the reference genome line). Using our filtered polymorphism data, we generated diversity summary statistics using custom python scripts across chromosome 2 in the sample of 178 C. grandiflora individuals (downsampled to 320 alleles, which allowed retention of 94.2% of sites) in 500-bp windows with 250-bp overlaps [57] or 50-SNP windows [58] . Linkage disequilibrium was calculated using Haploview [59] for unphased SNPs with minor allele frequency >5% in a 30-kb region centred around NPR1 , for all pairs of SNPs. Crossing experiments C. grandiflora × C. rubella crosses were generated by randomly crossing different C. grandiflora individuals originating from various Greek populations with several C. rubella accessions (see crossing scheme in Supplementary Fig. 7 ). The F1 plants were genotyped at the NPR1 and RPP5 loci. The NPR1 locus was genotyped using the primers oAS1129 and oAS1130 ( Supplementary Table 5 ). The deletion of RPP5 locus was genotyped using the primer pairs oAS839-oAS1133 and oAS839-oAS1276, while its presence was determined using the primer pairs oAS873 and oAS1123 ( Supplementary Table 5 ). The F2 progenies of these crosses were phenotyped for the segregation of the stunted growth phenotype and genotyped at NPR1 (primers oAS1129 and oAS1130), as well as at RPP5 using the very tightly linked molecular marker HiG2 to enable genotyping also for populations in which no RPP5 -presence allele segregated ( Supplementary Table 5 ). The marker HiG2 was chosen as it was the closest marker from RPP5 for which the underlying polymorphism was conserved between the different C. grandiflora and C. rubella parents used for the crosses. C. rubella 1504 × C. orientalis 1983 and C. orientalis 1983 × C. grandiflora 926 hybrids were obtained by ovule rescue as previously described [60] . Their F2 progenies were phenotyped and genotyped as indicated above. Transcriptome analysis Transcriptome sequencing was done for 99 samples from one C. grandiflora population, grown in a growth chamber at 22 °C with 16-h photoperiod. We extracted RNA using the Spectrum Plant Total RNA Kit (Sigma) from leaf tissue collected and flash frozen 5 weeks after germination. RNA was sequenced in two Illumina Hi-Seq flow cells with eight samples per lane. Reads were 100-bp long and paired end. We mapped RNA with Stampy 1.0.21 (ref. 61 ) to a custom reference genome constructed of exons and untranslated regions for each gene, using annotations from ref. 23 . Expression levels were measured as the number of paired fragments mapping to each gene using the HTSeq.scripts.count feature of HTSeq [62] , and read counts were normalized for sequencing depth by dividing each count by the median count for that individual. Genes with a median un-normalized expression level of <5 reads per individual or with very low variation in expression between individuals (coefficient of variation<0.1) were removed from further analysis leaving 18,692 genes in the analysis. Genes were linked to the NPR1 39-nt InDel genotype by testing for an association between NPR1 InDel genotype and gene-expression levels using a Kruskal–Wallis test, because expression data were not normally distributed. While none of the associations were significant after controlling for false discovery rates using Q value [63] , we included the 1,000 genes with the lowest P values for association in subsequent analyses. MapMan and MASTA analysis Identification of overrepresented gene categories within the 1,000 genes with the lowest P values for association with the NPR1 genotype was done using the MapMan ontology [39] and Fisher's exact test in R. The C. rubella MapMan mappings are available at http://mapman.gabipd.org . The same 1,000 genes were compared with the top 200 up- and downregulated genes of each experiment present in the MASTA data set of A. thaliana microarrays [40] . Only C. rubella genes with correspondence to A. thaliana microarray based on annotations in Phytozome version 8 (ref. 64 ) were considered, all other genes were filtered out from the MASTA data set. Top overlapping categories based on MASTA classification were determined using a Wilcoxon rank-sum test with overlap counts; P values were Bonferroni corrected for multiple testing. Statistical analysis Within each experiment, plants of the different genotypes were randomly assigned to positions in the trays, and trays were rotated once per week in the growth rooms. No blinding was performed. The statistical analysis was performed using R or Microsoft Excel 7. Data were presented as mean±s.e.m. To analyse the difference between genotypes Tukey’s honest significant difference test was carried out using agricolae package add-ons implemented in R software. To compare genotype frequencies between different phenotype classes, the χ 2 -test was used. P values<0.05 were considered statistically significant. Accession codes: Sequences of NPR1 and RPP5 alleles from the C. grandiflora × C. rubella RIL population have been deposited in NCBI GenBank nucleotide database under accession codes KT163438 to KT163440. Transcriptome and genome-resequencing data of C. grandiflora individuals have been deposited in NCBI under accession code PRJNA275635 . How to cite this article: Sicard, A. et al. Divergent sorting of a balanced ancestral polymorphism underlies the establishment of gene-flow barriers in Capsella . Nat. Commun. 6:7960 doi: 10.1038/ncomms8960 (2015).